EAT1 promotes tapetal cell death by regulating aspartic proteases during male reproductive development in rice Programmed cell death is essential for the development of multicellular organisms, yet pathways of plant programmed cell death and its regulation remain elusive. Here we report that ETERNAL TAPETUM 1, a basic helix-loop-helix transcription factor conserved in land plants, positively regulates programmed cell death in tapetal cells in rice anthers. eat1 exhibits delayed tapetal cell death and aborted pollen formation. ETERNAL TAPETUM 1 directly regulates the expression of OsAP25 and OsAP37 , which encode aspartic proteases that induce programmed cell death in both yeast and plants. Expression and genetic analyses revealed that ETERNAL TAPETUM 1 acts downstream of TAPETUM DEGENERATION RETARDATION, another positive regulator of tapetal programmed cell death, and that ETERNAL TAPETUM 1 can also interact with the TAPETUM DEGENERATION RETARDATION protein. This study demonstrates that ETERNAL TAPETUM 1 promotes aspartic proteases triggering plant programmed cell death, and reveals a dynamic regulatory cascade in male reproductive development in rice. In flowering plants, normal development of the anther, the specialized male reproductive organ, is essential to the alternation of life cycle between diploid sporophyte and haploid gametophyte generations. [1] , [2] Tapetal cells comprise the innermost anther wall layer, which encloses male reproductive cells, and undergo programmed cell death (PCD)-triggered degradation after the meiosis of microspore mother cells. This degradation process is essential for microspore development and pollen wall maturation; as a result, premature or delayed tapetal degradation causes male sterility. The tapetum is an excellent model system for investigating plant PCD [3] . Several transcriptional regulators have been reported to be associated with tapetal degeneration, including Arabidopsis MYB33/MYB65 [4] , DYSFUNCTIONAL TAPETUM1 (DYT1) [5] , DEFECTIVE IN TAPETAL DEVELOPMENT AND FUNCTION1 (TDF1) [6] , ABORTED MICROSPORE (AMS) [7] , MALE STERILITY1 [8] , rice GAMYB [9] , UNDEVELOPED TAPETUM1 [10] , TAPETUM DEGENERATION RETARDATION (TDR) [11] , PERSISTENT TAPETAL CELL 1 (PTC1) [12] , and APOPTOSIS INHIBITOR5 (API5) [13] . However, mechanisms by which these regulators regulate tapetal PCD remain unclear. PCD is crucial to the development and maintenance of multicellular organisms [14] . Some forms of plant PCD and animal apoptosis (one type of PCD) share several morphological and biochemical similarities, such as fragmentation of genomic DNA, presence of caspase-like proteolytic activities and cytochrome c release from the mitochondria [15] , [16] , [17] , [18] , [19] , [20] , [21] . In animals, cysteine aspartyl proteases (caspases) act as a core proteolytic component downstream of many PCD signal pathways [22] , [23] . Although caspase activities were detected in both animal and plant cells, plant genomes do not have apparent orthologous sequences of caspase genes [15] . Emerging evidence suggests that, in plants and yeast, a novel family of cysteine proteases called metacaspases appears to have endopeptidase activities and shares secondary structural homologies with mammalian caspases [24] , [25] , [26] , [27] , [28] , [29] . The single metacaspase Yeast Caspase-1 (YCA1) in yeast acts as a trigger in ageing and oxidative stress-activated PCD [24] . An Arabidopsis metacaspase, mcII-Pa, can cleave a phylogenetically conserved protein, Tudor staphylococcal nuclease, which is also the substrate of mammalian caspase-3, suggesting that some substrates in PCD are conserved between animals and plants [27] . Arabidopsis PBA1, one type of the β-subunit of the 20S proteasome, contributes to the caspase-3-like activity during defence response to bacteria in Arabidopsis [30] . In addition, aspartic protease is implicated in plant development and cell death. Arabidopsis UNDEAD , which encodes an A1 aspartic protease, suppresses tapetal PCD; knockdown of UNDEAD causes premature tapetal PCD [31] . Another Arabidopsis aspartic protease, PROMOTION OF CELL SURVIVAL1 (PCS1), has an anti-cell death role in embryonic and reproductive development [32] . A third Arabidopsis aspartic protease, CONSTITUTIVE DISEASE RESISTANCE 1 (CDR1) is associated with signalling in disease resistance [33] . S5 is the only characterized aspartic protease from rice; its gene is a major locus for indica–japonica hybrid sterility [34] . Despite these findings, how aspartic proteases function in plant PCD remains unknown at the mechanistic level. We previously reported that TDR, the rice ortholog of the Arabidopsis AMS protein, is a basic bHLH protein regulating tapetal PCD; tdr has expanded tapetal cells and delayed tapetal degeneration. Moreover, TDR is able to directly regulate the expression of a cysteine protease gene OsCP1 , yet the biochemical role of OsCP1 has not been characterized [11] . To address the mechanism underlying plant PCD and reveal additional regulators of the process, here we report the identification of ETERNAL TAPETUM 1 (EAT1), a key regulator of programmed tapetal development and degradation. Loss of function of EAT1 results in delayed tapetal PCD and aborted pollen development, causing complete male sterility. EAT1 encodes a putative bHLH transcription factor that directly regulates the expression of OsAP25 and OsAP37 , which encode aspartic proteases that promote cell death. Furthermore, EAT1 has the ability to interact with TDR. This work uncovers novel molecular pathways that determine programmed male reproductive development in plants. Identification and phenotypic analysis of the eat1 mutant To understand the mechanism underlying programmed male reproductive development in the model crop rice, we isolated a new male sterile mutant, eternal tapetum 1 ( eat1 ), from our rice mutant library made from an O. sativa ssp japonica cultivar, 9522 (ref. 35 ). The mutant exhibits normal vegetative development and female organ formation, but is completely male sterile and has shrunken anthers and aborted pollen grains ( Fig. 1a–h and Supplementary Fig. S1 ). All F1 plants of reciprocal crosses between the wild type and the mutant were fertile, and the F2 plants had an approximate 3:1 ratio for phenotypic segregation (fertility: sterility=160: 47, χ 2 =0.58, P >0.05, χ 2 test used), suggesting that this male sterile phenotype is caused by a single recessive mutation. 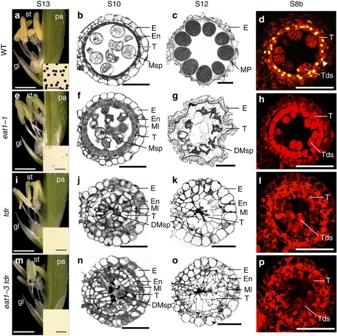Figure 1: Phenotypic analysis of anthers of the wild type and mutants. (a,e,i,m) Images of rice flowers and (insets) pollen grains stained by iodine-potassium iodide (I2-KI). Bars, 2 mm for the flowers and 200 μm for insets. (b,c,f,g,j,k,n,o) Transverse sections of anther locule (bars=50 μm); (d,h,l,p) TUNEL assays (bars, 50 μm). Red signal is PI staining, and yellow fluorescence is the merged signal from TUNEL (green) and PI. Arrow head points out the positive TUNEL signal. Bars, 50 μm. DMsp, degraded microspore; E, epidermis; En, endothecium; gl, glume; Ml, middle layer; MP, mature pollen; Msp, microspore; pa, palea; st, stamen; S8b, stage 8b; S10, stage 10; S12, stage 12; T, tapetum; Tds, tetrads. Figure 1: Phenotypic analysis of anthers of the wild type and mutants. ( a , e , i , m ) Images of rice flowers and (insets) pollen grains stained by iodine-potassium iodide (I 2 -KI). Bars, 2 mm for the flowers and 200 μm for insets. ( b , c , f , g , j , k , n , o ) Transverse sections of anther locule (bars=50 μm); ( d , h , l , p ) TUNEL assays (bars, 50 μm). Red signal is PI staining, and yellow fluorescence is the merged signal from TUNEL (green) and PI. Arrow head points out the positive TUNEL signal. Bars, 50 μm. DMsp, degraded microspore; E, epidermis; En, endothecium; gl, glume; Ml, middle layer; MP, mature pollen; Msp, microspore; pa, palea; st, stamen; S8b, stage 8b; S10, stage 10; S12, stage 12; T, tapetum; Tds, tetrads. Full size image To characterize the cellular abnormality of eat1-1 during male reproductive development, anther transverse sections were examined. Similar to the wild type, the eat1-1 mutant anthers appeared to undergo normal meiosis, forming tetrads of haploid microspores at late stage 8 (stage 8b) ( Supplementary Fig. S2 ). Consistent with this observation, normal chromosome separation during meiosis and regular tetrads could be seen in eat1-1 microspore mother cells, as revealed by 4′,6-diamidino-2-phenylindole staining ( Supplementary Fig. S3a ). After stage 10, the wild-type tapetal cells had condensed cytoplasm, then became thinner and were eventually degenerated before mature pollen grains were formed ( Fig. 1b and c and Supplementary Fig. S2a ). In contrast, the eat1-1 mutant had thicker and darkly stained tapetal cells ( Fig. 1f ), and abnormal abortion of the anther locule and microspores ( Fig. 1g and Supplementary Fig. S2b ). These results together show that in the eat1 mutant, anther development and microspore formation are aborted. eat1 exhibits delayed tapetal PCD The cellular analysis described above suggests that EAT1 may affect the degradation of tapetal cells. In plants, tapetal cell degeneration is triggered by PCD, which is characterized by cell condensation, nuclear degeneration and membrane breakdown, and the cleavage of nuclear DNA [11] . To test whether the eat1 mutant anthers are defective in tapetal PCD, we performed the terminal deoxynucleotidyl transferase-mediated dUTP nick-end labeling (TUNEL) assay and transmission electron microscopy (TEM). Consistent with our previous observations [11] , the TUNEL-positive signal in wild-type tapetal cells commenced at stage 8 during late meiosis, became intense at stage 9 when the microspore is released from the tetrad, and weakened at stage 12 when mature pollen grains are formed ( Fig. 1d and Supplementary Fig. S3b ). However, no obvious DNA fragmentation signal was observed in eat1 tapetal cells till stage 10, when the vacuolated microspore forms ( Fig. 1h and Supplementary Fig. S3b ). At stage 11 during mitosis I, weak DNA fragmentation signal was seen in all four layers of the eat1 anthers ( Supplementary Fig. S3b ), suggesting delayed and abnormal PCD. In agreement with results of the TUNEL assays, TEM analysis also revealed a delay in PCD in the mutant ( Fig. 2a–h ). At stage 10, the wild-type tapetal cells showed typical signs of PCD, such as condensed cytoplasm and the presence of poorly defined organelles ( Fig. 2a ). In contrast, eat1-1 tapetal cells contained abundant distinctive organelles, including the endoplasmic reticulum (ER), Golgi apparatus, a large number of ribosomes attached to the rough-surfaced ER, and an increased number of enlarged mitochondria ( Fig. 2b ), suggesting the retention of highly active metabolism and/or delayed cell death processes in the tapetum. At stage 11, the wild-type tapetal cells became more degenerated with the breakage of the nuclear membrane ( Fig. 2c ). By contrast, at this stage, the eat1-1 tapetal cells appeared less disintegrated, with intact nuclear membranes and increased number of mitochondria and vacuoles ( Fig. 2d ). 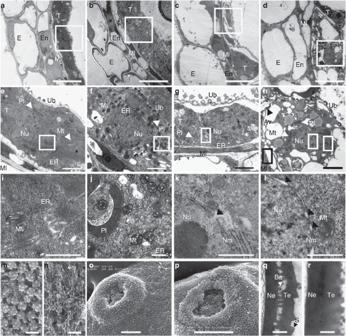Figure 2: Electron micrographs of anthers and pollen grains. The transverse section of anthers at early stage 10 (10a) (a,b) and stage 11 (c,d). The tapetal cells of stage 10a (e,f) and stage 11 (g,h) are high magnifications of the insets of (a–d). (i,j) Higher magnification of the insets of (e,f) showing mitochondria (Mt) and endoplasmic reticulum (ER). (k,l) Higher magnification of the insets of (g,h) showing the nuclear membranes. (k) Disintegration of the wide-type nuclear membrane, where the breakage is marked by the black arrowhead. (l) Theeat1-1nuclear membrane was intact and partially widened, marked by the black arrowhead. (m–p) Scanning electron microscopic analysis of the inner surface of the tapetal layer (m,n) and pollen grains (o,p) at stage 10. (q–r) Transverse section of the exine of microspore wall at stage 11, showing tectum, nexine, bacula (white arrow head) and spine distribution on the exine. (a,c,e,g,i,k,m,o,q) Wild type. (b,d,f,h,j,l,n,p,r)eat1-1. Bars, 5 μm in (a–d), 2 μm in (e–h,o,p) and 500 nm in (i–n,q,r). (e,f,g,h,j,k,l) Were high. As, abnormal secretion; Av, abnormal vacuole; Ba, bacula; E, epidermis; En, endothecium; Ml, middle layer; Mt, mitochondria; Ne, nexin; Nm, Nuclear membranee; Nu, nucleus; Pl, plastid; S, spine; T, tapetum; Te, tectum; Ub, ubisch body. Figure 2: Electron micrographs of anthers and pollen grains. The transverse section of anthers at early stage 10 (10a) ( a , b ) and stage 11 ( c , d ). The tapetal cells of stage 10a ( e , f ) and stage 11 ( g , h ) are high magnifications of the insets of ( a – d ). ( i , j ) Higher magnification of the insets of ( e , f ) showing mitochondria (Mt) and endoplasmic reticulum (ER). ( k , l ) Higher magnification of the insets of ( g , h ) showing the nuclear membranes. ( k ) Disintegration of the wide-type nuclear membrane, where the breakage is marked by the black arrowhead. ( l ) The eat1-1 nuclear membrane was intact and partially widened, marked by the black arrowhead. ( m – p ) Scanning electron microscopic analysis of the inner surface of the tapetal layer ( m , n ) and pollen grains ( o , p ) at stage 10. ( q – r ) Transverse section of the exine of microspore wall at stage 11, showing tectum, nexine, bacula (white arrow head) and spine distribution on the exine. ( a , c , e , g , i , k , m , o , q ) Wild type. ( b , d , f , h , j , l , n , p , r ) eat1-1 . Bars, 5 μm in ( a – d ), 2 μm in ( e – h , o , p ) and 500 nm in ( i – n , q , r ). ( e , f , g , h , j , k , l ) Were high. As, abnormal secretion; Av, abnormal vacuole; Ba, bacula; E, epidermis; En, endothecium; Ml, middle layer; Mt, mitochondria; Ne, nexin; Nm, Nuclear membranee; Nu, nucleus; Pl, plastid; S, spine; T, tapetum; Te, tectum; Ub, ubisch body. Full size image Ubisch bodies are unique structures observed in cereals and other plants, which are proposed to function in exporting tapetum-produced lipidic sporopollenin precursors across the hydrophilic cell wall to the locule for the formation of the lipidic microspore exine [36] , [37] , [38] . At stage 10, the internal surface of the wild-type tapetum contained abundant Ubisch bodies ( Fig. 2e and m ). In eat1-1 , however, the Ubisch bodies were abnormally round-shaped and covered by a layer of tubular structures ( Fig. 2f and n ). As a result, eat1-1 displayed irregular pollen exine patterning, such as no obvious inter-layer space between the nexine (foot layer) and tectum ( Fig. 2o–r ). These observations collectively suggest that EAT1 has a key role in tapetal PCD, a process required for microspore development. EAT1 encodes a tapetum-expressed bHLH transcription factor Map-based cloning was used to identify the EAT1 gene. Using 120 mutant individuals from the F2 population of a cross between eat1 -1 and Guang Lu Ai (an indica variety), the EAT1 gene was mapped to chromosome 4 between XY409-4 and XY409-5, two Insertion-Deletion markers that define a 3-cM (centimorgan) DNA region ( Fig. 3a ). While sequencing anther-expressed candidate genes within this region, we found deletions of the 543rd and 544th nucleotides (T and G) in the coding region of a gene that corresponded to LOC_Os04g51070 ( http://www.gramene.org/ , also annotated as Os04g0599300 by http://rapdb.dna.affrc.go.jp/ ) ( Fig. 3b ). From the Tos17-insertion mutant library (Rice Genome Resource Center, RGRC), we later identified two additional alleles, eat1-2 and eat1-3 ( Fig. 3b and Supplementary Fig. S1e ), both of which also showed male sterility ( Supplementary Fig. S1a–d ) and delayed cell death in the tapetum ( Supplementary Fig. S3b ). 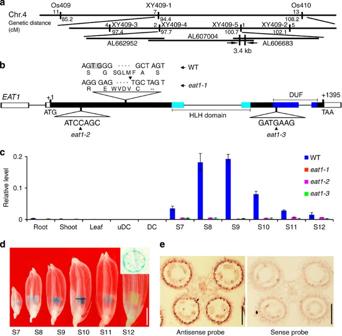Figure 3: Identification and expression analyses ofEAT1. (a) Fine mapping ofeat1-1to chromosome 4. Names and positions of the molecular markers are indicated. AL662952, AL607004 and AL606683 are rice genomic DNA accession numbers of bacterial artificial chromosome clones. (b) A schematic representation ofEAT1. (c)EAT1expression analysis by qRT–PCR. One-way analysis of variance test was used. Results are presented as mean±s.e. (d) GUS staining of transgenic anthers containingEAT1pro:GUS; bar, 2 mm. Inset, GUS staining in a transverse section of a stage 10 anther locule (as indicated by the black horizontal bar); bar, 50 μm. (e)In situanalysis ofEAT1in wide-type anthers at stage 8. Bars, 50 μm. uDC, undifferentiated callus; DC, differentiating callus; S7 to 12, Stage 7 to 12. Figure 3: Identification and expression analyses of EAT1 . ( a ) Fine mapping of eat1-1 to chromosome 4. Names and positions of the molecular markers are indicated. AL662952, AL607004 and AL606683 are rice genomic DNA accession numbers of bacterial artificial chromosome clones. ( b ) A schematic representation of EAT1 . ( c ) EAT1 expression analysis by qRT–PCR. One-way analysis of variance test was used. Results are presented as mean±s.e. ( d ) GUS staining of transgenic anthers containing EAT1 pro : GUS ; bar, 2 mm. Inset, GUS staining in a transverse section of a stage 10 anther locule (as indicated by the black horizontal bar); bar, 50 μm. ( e ) In situ analysis of EAT1 in wide-type anthers at stage 8. Bars, 50 μm. uDC, undifferentiated callus; DC, differentiating callus; S7 to 12, Stage 7 to 12. Full size image We further investigated the spatio-temporal expression pattern of the EAT1 gene by qualitative and quantitative RT–PCR (qRT–PCR) analyses. In the wild type, EAT1 is weakly expressed in roots, shoots and leaves, and highly expressed in the anther from stage 7 to 12, while a dramatic reduction in expression was detected in the anthers in all three eat1 alleles ( Fig. 3c ). In GUS-stained EAT1 pro : GUS transgenic flowers, GUS signals started to appear in anthers at stage 7, became stronger from stage 8 to 9, and were nearly undetectable at stage 12 ( Fig. 3d ). Further transverse section analysis of GUS-stained locules and in situ RNA hybridization indicated that EAT1 is highly expressed in the tapetum ( Fig. 3d and e ). Previous studies suggested that tapetal PCD is initiated at stage 8 during the meiosis of microspore mother cells [11] , thus the spatio-temporal expression pattern of EAT1 is in good agreement with a potential role of this protein in tapetal PCD. EAT1 acts downstream from and interacts with TDR To understand the role of EAT1 in the regulatory network of tapetal development, the expression level of several genes encoding transcriptional regulators or Leu-rich repeat receptor-like protein kinase in this process was examined by qRT–PCR. Genes such as MULTIPLE SPOROCYTE ( MSP1 ) [39] , GAMYB [9] , UDT1 [10] , TDR [11] , PTC1 [12] , and API5 [13] showed no obvious changes in eat1-1 anthers ( Supplementary Fig. S4a–f ). OsCP1 , a cysteine protease-encoding gene [40] that is directly regulated by TDR and API5 [11] , [13] , exhibited a slight reduction in expression until stage 10, and an increase in expression after stage 11 ( Supplementary Fig. S4g ). Conversely, the expression of EAT1 was slightly decreased in gamyb1–4 and udt1 , and greatly reduced in tdr and ptc1 ( Supplementary Fig. S4h ), suggesting that TDR and PTC1 may positively regulate the expression of EAT1 . Previously we showed that TDR is a positive transcriptional regulator in tapetal PCD [11] . To determine the relationship between EAT1 and TDR , we constructed the eat1-3 tdr double mutant. Histological analyses showed that eat1-3 tdr displayed defective anther development, including delayed tapetal degeneration, enormously expanded tapetal cells and negative TUNEL signal ( Fig. 1m–p and Supplementary Fig. S3b ), similar to the phenotype of tdr ( Fig. 1i–l and Supplementary Fig. S3b ). We thus propose that EAT1 functions in one of the pathways controlled by TDR and that TDR may regulate the expression of EAT1 . Our previous studies showed that two Arabidopsis bHLH proteins, AtbHLH089 and AtbHLH091, interact with AMS, the ortholog of TDR in Arabidopsis [7] . EAT1 shares sequence similarity with AtbHLH089 and AtbHLH091 [41] . To gain further insight into the function of EAT1, we performed a yeast two-hybrid analysis to determine whether EAT1 interacts with TDR. Yeast strains coexpressing EAT1 and TDR grew normally under stringent selection conditions (30 mM 3-amino-1, 2, 4-triazole) and displayed activation of the expression of HIS3 , ADE2 and the LacZ reporter genes, confirming the interaction between EAT1 and TDR ( Fig. 4a ). In vitro interaction between these two proteins was further confirmed using co-immunoprecipitation (Co-IP) assays ( Fig. 4b ). Furthermore, we validated this interaction using bimolecular fluorescent complementation (BiFC) in rice protoplasts. In contrast to the negative control, yellow fluorescent protein (YFP) signals were observed in the nucleus of the cells expressing EAT-nYFP and TDR-cYFP ( Fig. 4c ), confirming the interaction of the two proteins in vivo . In support of these data, TDR is also highly expressed in the tapetum [11] . 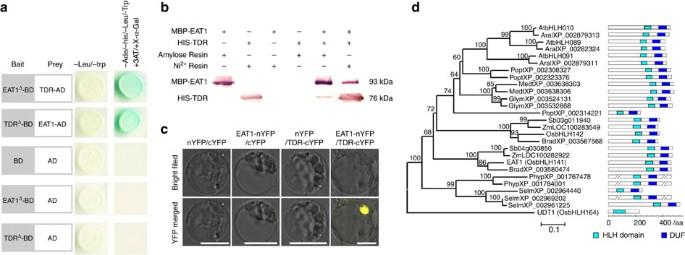Figure 4: EAT1 interacts with TDR and phylogenic analysis ofEAT1. (a) EAT1 and TDR interact in yeast cells. Co-expression of EAT1 and TDR was able to activate the expression of theHIS3,ADE2andLacZreporter genes. (b) Co-IP of MBP-EAT1 and HIS-TDR recombinant proteins expressed inE. coli. Maltose-binding protein (MBP) alone and HIS alone were used as negative controls. (c) BiFC in rice protoplasts expressing the indicated constructs. Bars, 10 μm. (d) A neighbour-joining tree of EAT1 and its homologues. Aral,Arabidopsis lyrata;At,Arabidopsis thaliana; Brad,Brachypodium distachyon;Glym,Glycine max; Medt,Medicago truncatula; Os,Oryza Sativa; Phyp,Physcomitrella patens; Popt,Populus trichocarpa;Sb,Sorghum bicolours; Selm,Selaginella moellendorffii; Zm,Zea may. Figure 4: EAT1 interacts with TDR and phylogenic analysis of EAT1 . ( a ) EAT1 and TDR interact in yeast cells. Co-expression of EAT1 and TDR was able to activate the expression of the HIS3 , ADE2 and LacZ reporter genes. ( b ) Co-IP of MBP-EAT1 and HIS-TDR recombinant proteins expressed in E. coli . Maltose-binding protein (MBP) alone and HIS alone were used as negative controls. ( c ) BiFC in rice protoplasts expressing the indicated constructs. Bars, 10 μm. ( d ) A neighbour-joining tree of EAT1 and its homologues. Aral, Arabidopsis lyrata; At, Arabidopsis thaliana ; Brad, Brachypodium distachyon; Glym, Glycine max ; Medt, Medicago truncatula ; Os, Oryza Sativa ; Phyp, Physcomitrella patens ; Popt, Populus trichocarpa; Sb, Sorghum bicolours ; Selm, Selaginella moellendorffii ; Zm, Zea may . Full size image EAT1 is conserved in terrestrial plants To understand the evolution of EAT1 , we used the full-length EAT1 protein sequence to search available public databases and retrieved a total of 26 homologues from 10 diverse plant species from moss, pteridophytes, to angiosperms ( Fig. 4d and Supplementary Tables S1 and S2 ). The molecular functions of these homologues have not been reported. Phylogenetic analysis showed that EAT1 and the 26 homologues each have a single HLH domain and a conserved but previously uncharacterized motif at the C-terminus, designated as DUF for D omain of U nknown F unction ( Figs 3b and 4d and Supplementary Fig. S5 and Table S2 ). Moreover, EAT1 and three homologues from Sorghum bicolour (Sb04g030850), Zea mays (ZmLOC100282922) and Brachypodium distachyon (BradXP_003580474), respectively, were grouped in a subclade ( Fig. 4d ), suggesting that EAT1 and its homologues underwent diversification during grass evolution. EAT1 has one homologue from rice (OsbHLH142), which shares 40.8% identity with EAT1 in the HLH and DUF domains, and three homologues from Arabidopsis (AtbHLH091, AtbHLH089, AtbHLH010), which share an average of ~40% identity with EAT1 in these two conserved domains ( Fig. 4d and Supplementary Fig. S5 ). In addition, seven of the EAT1 homologues identified from Medicago truncatula , Populus trichocarpa , Glycine max , Arabidopsis and rice are also expressed in reproductive organs, such as inflorescences and male organs ( Supplementary Table S1 ). These findings suggest a specific and possibly conserved role for EAT1 in male reproductive development in plants. EAT1 directly regulates the expression of aspartic proteases To understand the mechanism of EAT1 ’s function in gene expression during tapetal PCD and microspore development, we performed microarray analysis of eat1 at stage 9 of anther development, and observed changes in the expression of many genes (data not shown). Among them, two aspartic protease-encoding genes, OsAP25 and OsAP37 , showed a significant reduction in expression, which was further confirmed by qRT–PCR ( Fig. 5a and Supplementary Fig. S6a and b ). Interestingly, the expression of these two genes is also greatly reduced in tdr ( Supplementary Fig. S6b ), the mutant of another transcription factor involved in rice tapetal PCD [11] (see previous section). Therefore, we chose to focus on OsAP25 and OsAP37 to determine whether these genes are directly regulated by EAT1 in PCD. 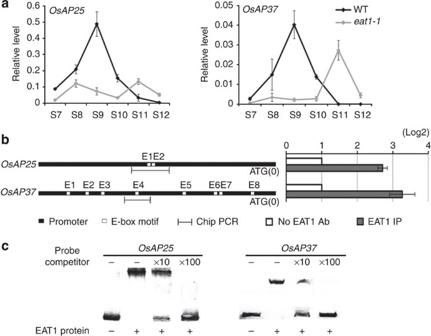Figure 5: Analysis of genes regulated byEAT1. (a) qRT–PCR analysis ofOsAP25andOsAP37. (b) Presence of the E-box motifs in the promoters ofOsAP25andOsAP37(left) and qChIP-PCR results (right) showing preferred binding of EAT1 to the promoter fragments containing the E-box motifs, that is, E1E2 onOsAP25and E4 onOsAP37. (c) EMSA assay showing the binding of recombinant EAT1 to the promoter fragments ofOsAP25andOsAP37. The binding complex could be outcompeted by increasing quantities of unlabelled DNA fragments ( × 10 and × 100 of unlabelled DNA fragments). One-way analysis of variance test was used. Results are presented as mean±s.e. E(n), E-box motif; EAT1 IP, immunoprecipitated chromatin by EAT1 antibody; No EAT1 Ab, negative control without EAT1 antibody; S7 to 12, Stage 7 to 12. Figure 5: Analysis of genes regulated by EAT1 . ( a ) qRT–PCR analysis of OsAP25 and OsAP37 . ( b ) Presence of the E-box motifs in the promoters of OsAP25 and OsAP37 (left) and qChIP-PCR results (right) showing preferred binding of EAT1 to the promoter fragments containing the E-box motifs, that is, E1E2 on OsAP25 and E4 on OsAP37 . ( c ) EMSA assay showing the binding of recombinant EAT1 to the promoter fragments of OsAP25 and OsAP37 . The binding complex could be outcompeted by increasing quantities of unlabelled DNA fragments ( × 10 and × 100 of unlabelled DNA fragments). One-way analysis of variance test was used. Results are presented as mean±s.e. E(n), E-box motif; EAT1 IP, immunoprecipitated chromatin by EAT1 antibody; No EAT1 Ab, negative control without EAT1 antibody; S7 to 12, Stage 7 to 12. Full size image Given that bHLH transcription factors are predicted to regulate gene expression by binding to the E-box (CANNTG) in the promoter of target genes [7] , we used chromatin immunoprecipitation (ChIP)-PCR and electrophoretic mobility shift assay (EMSA) assays to test whether EAT1 could directly regulate OsAP25 and OsAP37 . EAT1 polyclonal antibodies were generated using an EAT1-specific peptide fragment (see Methods), and their specificities were confirmed using protein gel blot analysis ( Supplementary Fig. S7a ) before the antibodies were used in ChIP-PCR. Results from ChIP-PCR and EMSA demonstrated that EAT1 binds to the E-box-containing promoters of OsAP25 and OsAP37 ( Fig. 5b and c ). In contrast, we did not observe an obvious association of EAT1 with the promoter of the control gene OsAP19 , which only displayed a slight reduction in expression in eat1-1 ( Supplementary Fig. S7b and c ). These data suggest that EAT1 directly regulates the expression of these two aspartic protease genes. Consistent with a role of EAT1 in regulating OsAP25 and OsAP37 , all three genes were highly expressed in tapetal cells ( Fig. 3c–e and Fig. 5a and Supplementary Fig. S6c ). One tissue in which EAT1 and OsAP25 were differentially expressed was the callus, where OsAP25 transcripts were observed yet no EAT1 expression signals were seen, suggesting a possible separate role for OsAP25 in rice regeneration ( Fig. 3c and Supplementary Fig. S6a ). In agreement with this hypothesis, we were unable to use the artificial microRNA technology to obtain transgenic plants via calli to suppress the expression of OsAP25 (data not shown). OsAP25 and OsAP37 activate cell death in yeast To characterize the potential role of OsAP25 and OsAP37 in PCD, GAL10 promoter-driven OsAP25 and OsAP37 were individually transformed into a PCD-deficient yeast strain, Δyca1 [23] . After 4-h 20 mM H 2 O 2 treatment, 82% and 71% of the yeast cells overexpressing OsAP25 and OsAP37 , respectively, displayed positive signals when labelled with the mammalian caspase substrate FITC-VAD-fmk, suggesting that OsAP25 and OsAP37 share a similar function with YCA1 in promoting PCD process in yeast ( Fig. 6a ). Eight hours after the H 2 O 2 treatment, propidium iodide (PI) staining and flow cytometry analysis were performed to measure the number of live cells. Whereas 93% of the non-transformed Δyca1 cells were still alive, cells overexpressing OsAP25 and OsAP37 had a survival rate of 18% and 29%, respectively ( Fig. 6b ). These findings suggest that, similar to the yeast metacaspase protein YCA1 [24] , OsAP25 and OsAP37 have the ability to promote cell death in yeast cells. 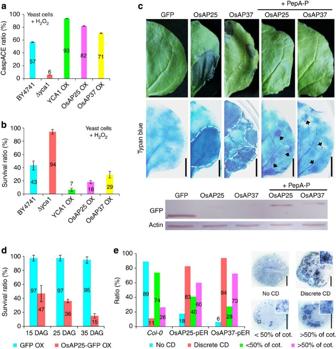Figure 6: OsAP25 and OsAP37 promote PCD in yeast and plants. (a) FITC-VAD-fmk staining showing caspase activities in yeast strains. (b) Survival rates of yeast cells overexpressingOsAP25andOsAP37as shown by PI staining. (c) Tobacco leaves transiently expressingGFP,OsAP25-GFPorOsAP37-GFPand were stained by Trypan blue. The dead epidermal cells are indicated by dashed lines and arrows. Bars, 1 cm. Below the leaf images is the western blot analysis of extracts of tobacco leaves transiently expressingGFP,OsAP25-GFPorOsAP37-GFP, using the GFP antibody. (d) Survival rates ofArabidopsisseedlings overexpressingOsAP25-GFP, 15, 25 and 35 days after germination. (e) Quantification of Trypan blue staining in leaves and cotyledons of transgenic seedlings expressing oestrogen-inducedOsAP25(OsAP25-pER) orOsAP37(OsAP37-pER) 48 h after estradiol treatment. Bars, 1 mm. The insets are higher magnifications of the boxed regions.n=78 for cotyledons and 80 for leaves. One-way analysis of variance test was used. Results are presented as mean±s.e. CD, cell death of leaf; DAG, days after germination; discrete CD, dotted distribution of cell death on the leaf; NO CD, no cell death detected; PepA-P, Pepstatin A; <50% of cot., extensive cell death covering <50% of the cotyledon; >50% of cot., extensive cell death covering >50% of the cotyledon. Figure 6: OsAP25 and OsAP37 promote PCD in yeast and plants. ( a ) FITC-VAD-fmk staining showing caspase activities in yeast strains. ( b ) Survival rates of yeast cells overexpressing OsAP25 and OsAP37 as shown by PI staining. ( c ) Tobacco leaves transiently expressing GFP , OsAP25-GFP or OsAP37-GFP and were stained by Trypan blue. The dead epidermal cells are indicated by dashed lines and arrows. Bars, 1 cm. Below the leaf images is the western blot analysis of extracts of tobacco leaves transiently expressing GFP , OsAP25-GFP or OsAP37-GFP , using the GFP antibody. ( d ) Survival rates of Arabidopsis seedlings overexpressing OsAP25-GFP , 15, 25 and 35 days after germination. ( e ) Quantification of Trypan blue staining in leaves and cotyledons of transgenic seedlings expressing oestrogen-induced OsAP25 ( OsAP25-pER ) or OsAP37 ( OsAP37-pER ) 48 h after estradiol treatment. Bars, 1 mm. The insets are higher magnifications of the boxed regions. n =78 for cotyledons and 80 for leaves. One-way analysis of variance test was used. Results are presented as mean±s.e. CD, cell death of leaf; DAG, days after germination; discrete CD, dotted distribution of cell death on the leaf; NO CD, no cell death detected; PepA-P, Pepstatin A; <50% of cot., extensive cell death covering <50% of the cotyledon; >50% of cot., extensive cell death covering >50% of the cotyledon. Full size image Overexpression of OsAP25/37 leads to cell death in plants To further test the roles of the aspartic proteases in cell death, we expressed the full-length CDS of OsAP25 or OsAP37 driven by the CAMV 35S promoter in plants. Trypan blue vital staining of tobacco leaves revealed substantially increased death of epidermal and mesophyll cells in leaves transiently expressing OsAP25 or OsAP37 compared with those expressing green fluorescent protein (GFP), or OsAP25 and OsAP37 together with the aspartic protease-specific inhibitor pepstatin A (penetratin, PepA-P) ( Fig. 6c ). Furthermore, overexpression of OsAP25-GFP in Arabidopsis caused the death of 53% of the transgenic seedlings 15 days after seed germination and left ~85% of the plants dead by 35 days ( Fig. 6d ). No stable transgenic lines overexpressing OsAP37 were obtained, indicating that overexpression of OsAP37 may block early plant development or cause premature death. Consistent with these results, Arabidopsis transgenic lines expressing inducible OsAP25 or OsAP37 exhibited extensive cell death (indicated by Trypan blue staining) in leaves and cotyledons 48 h after their gene expression was induced by estradiol ( Fig. 6e ). In this study, we have revealed an essential role of EAT1 in programmed tapetal cell death and pollen formation in the monocot crop rice. By in vivo and in vitro analyses, we show that EAT1 directly regulates the expression of two aspartic protease genes that promote cell death in yeasts and plants. Additionally, genetic and molecular analyses suggest that EAT1 acts downstream of TDR in triggering cell death, and that EAT1 can also form a protein complex with TDR. These findings suggest that EAT1 and TDR represent two key factors in the regulatory network of anther development in rice and that one pivotal role for EAT1 is to regulate the expression of aspartic protease genes. Both plant and yeast cells have morphological and biochemical PCD features similar to that of animal apoptosis. Furthermore, plant cell death can be blocked by human caspase inhibitors, and caspase-like activities were detected in plants [18] , [19] , [20] , [21] , [30] , [42] . In this study, we showed that two aspartic proteases, OsAP25 or OsAP37, can rescue the yeast metacaspase-deficient strain, Δyca1 . Ectopic expression of OsAP25 or OsAP37 promotes cell death in plants as well, and treatment with aspartic protease-specific inhibitor significantly reduced this effect. These results suggest that a subset of plant aspartic proteases also function as executors in PCD, indicating possible mechanistic similarities between apoptosis in animals and PCD in yeast and plants. However, although yeast metacapase mutant strains expressing OsAP25 or OsAP37 could be labelled by the caspase substrate FITC-VAD-fmk ( Fig. 6a ), we were unable to detect caspase-1-9 activities in mammalian cell extracts expressing OsAP25 or OsAP37 (data not shown). This result may reflect the fact that these aspartic proteases have target proteins or cleavage motif distinct from animal caspases. Although YCA1 was initially reported to have caspase-like activity [24] , subsequent studies showed that Arabidopsis metacaspases AtMCP1b and AtMCP2b, as well as yeast YCA1, exhibit arginine/lysine-specific endopeptidase activities with no direct cleavage activity on caspase-specific substrates [25] , suggesting that the metacaspases may activate downstream effective caspase-like protease(s) involved in cell death [25] . Consistent with this, crystal structure analysis revealed that even though the YCA1 metacaspase has a caspase-like fold, the protein exists as a monomer both in solution and in crystals, instead of forming homodimers like canonical caspases [29] . We thus propose that OsAP25 and OsAP37 may activate downstream caspase-like protease(s) involed in PCD rather than directly acting on caspase-specific substrates. Moreover, even though OsAP25, OsAP37, PCS1 and UNDEAD belong to the C-group of aspartic proteases [43] , [44] , OsAP25 and OsAP37 can promote cell death ( Fig. 6b–e ) whereas UNDEAD and PCS1 have anti-PCD functions [31] , [32] , suggesting diversified roles of aspartic proteases in plant PCD. Additionally, OsAP25 and OsAP37 display reduced expression in udt1 , tdr and ptc1 , mutants with delayed tapetal PCD ( Supplementary Fig. S6b ), further supporting the role of these two aspartic proteases in tapetal PCD. How UDT1 and PTC1 affect the expression of OsAP25 and OsAP37 remains to be elucidated. In this study, we show that EAT1 has a unique regulatory role in tapetal PCD in comparison with previously identified proteins involved in tapetal degeneration. Unlike the expanded tapetal cells in gamyb , udt1 and tdr [9] , [10] , [11] , or necrosis in ptc1 tapetum [12] , eat1-1 displays a delay in tapetal PCD without cell enlargement or necrosis-like phenotypes ( Fig. 1a–l and Fig 2 and Supplementary Figs S2 and 3b ). We speculate that GAMYB, UDT1 and TDR have additional roles in modulating tapetal cell size besides their roles in tapetal PCD, while the major role of EAT1 is to positively regulate tapetal PCD. Although EAT1 interacts with TDR, TDR is unable to bind to the promoters of OsAP25 and OsAP37 , and EAT1 cannot bind to the promoter of OsCP1 , a direct target of TDR [11] (data not shown). These results suggest that EAT1 and TDR may have diversified roles in the regulatory network in anther development. Furthermore, the expression of EAT1 is obviously reduced in tdr ( Supplementary Fig. S4h ), and eat1 tdr double mutants exhibit the expanded tapetal cells similar to tdr ( Fig. 1i–p ), suggesting that EAT1 acts downstream of TDR in regulating tapetal PCD. Consistent with this, the expression of OsAP25 and OsAP37 is greatly reduced in tdr ( Supplementary Fig. S6b ). It seems that EAT1 is directly regulating PCD via aspartic proteases and TDR’s role in PCD is, at least in part, through EAT1 ( Fig. 7 ). 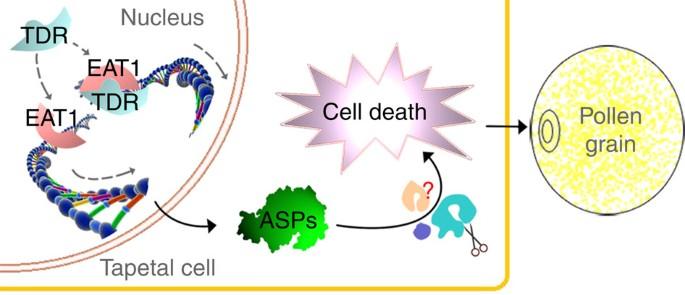Figure 7: A proposed model for the role of EAT1 in tapetal PCD. EAT1 acts downstream of TDR in the nucleus. EAT1 directly promotes the expression ofOsAP25andOsAP37(ASPs), which encode aspartic proteases triggering the tapetal PCD to affect tapetal development and pollen formation. Figure 7: A proposed model for the role of EAT1 in tapetal PCD. EAT1 acts downstream of TDR in the nucleus. EAT1 directly promotes the expression of OsAP25 and OsAP37 ( ASPs ), which encode aspartic proteases triggering the tapetal PCD to affect tapetal development and pollen formation. Full size image EAT1 homologues are present in land plants and are possibly involved in male reproductive development because of their expression patterns ( Supplementary Table S1 ). We propose that EAT1 and its close homologues have played a crucial role in land plant colonization, possibly through their involvement in the formation of the male gamete. To date, functions of EAT1 homologues have not been reported. Our work therefore provides a clue to the possible roles of these transcriptional factors in plant programmed male development across diverse plant species. In summary, this work has uncovered a previously unknown molecular pathway that controls programmed male reproductive development in plants, as depicted in a working model ( Fig. 7 ). Given the importance of rice as a major crop, this finding may provide molecular basis for rational manipulation of pollen fertility to improve crop yield. Mutant identification and molecular and phenotypic analyses Mutant identification, plant growth, map-based cloning, phenotypic characterizations and gene expression analyses were performed using methods from our previous reports [7] , [11] , [12] . Anther staging is defined by Zhang and Wilson [45] . To fuse the EAT1 promoter with the GUS (β-glucuronidase) reporter gene, a 2,102-bp fragment upstream from the start codon of EAT1 was amplified from wild-type rice genomic DNA and cloned into the binary vector pCAMBIA1301 . For in situ analysis of EAT1 , OsAP25 and OsAp37 , a 491-bp EAT1 fragment was amplified from the EAT1 cDNA clone (AK119509, provided by RGRC); a 346-bp OsAP25 - and a 362-bp OsAP37 -specific fragment were amplified from wild-type rice genomic DNA. The resultant DNA fragments were cloned into pBlueScript II SK ( pBSK ) for producing the RNA hybridization probes. Yeast two-hybrid assay The MATCHMAKER GAL4 Two-Hybrid System (Clontech) was used. Because both full-length EAT1 and TDR proteins were observed to self-activate, we made a truncated EAT1, which contains the C-terminal bHLH domain (EAT1 Δ , amino acids 255–464), and a truncated TDR containing the N-terminal bHLH domain (TDR Δ , amino acids 1–344). The full-length EAT1 and TDR were cloned into pGAD-T7 (Clontech), and EAT1 Δ and TDR Δ were cloned into pGBK-T7 (CLONTECH), respectively. His and Ade selection and X-α-Gal filter assay were performed according to the manufacturer’s instructions. Co-immunoprecipitation Recombinant EAT1 expressed in pMAL-c2X and TDR expressed in pET32a (HIS-tag, Novagen) were purified using the amylose and Ni 2+ resin, respectively. The eluent was analysed using 10% SDS–polyacrylamide gel electrophoresis, and tested using the monoclonal antibodies against maltose-binding protein (NEB, E8032) and HIS (Beyotime, AH367). Bimolecular fluorescence complementation The N-terminal 155 amino acids of nYFP was translationally fused to the C-terminus of full-length EAT1. The C-terminal 84 amino acids of YFP (cYFP) was translationally fused to the C-terminus of full-length TDR. The procedure of BiFC was described in Schütze et al. [46] Phylogenetic analysis Multiple alignments were performed using Muscal 3.6 ( http://www.ebi.ac.uk/Tools/msa/muscle/ ). A phylogenetic tree was constructed with the aligned sequences from the region from the HLH to the DUF domain (correlating to amino acids 251–464 on EAT1). MEGA (version 3.0) [47] and the Neighbor-Jointing (NJ) methods were used with p-distance model and pairwise deletion and bootstrap (1000 replicates; random seed). The Max Parsimony method of MEGA was also used to support the NJ tree, using the default parameter. qChIP-PCR To generate EAT1 antibodies, a DNA fragment encoding an EAT1-specific peptide (amino acids 1–109) was cloned into the bacterial expression vector pGEX-6P-1 (GE Healthcare, Cardiff, UK). The EAT1-specific peptide fused with glutathione S -transferase (GST) was expressed according to the manufacturer’s instructions, and used to generate an EAT1-specific polyclonal antibody, using methods described in Huang et al. [48] The specificity of the EAT1 antibody was examined using the method described by Zhang et al. [49] To express the EAT1 protein, a fragment containing the C-terminal 266 aa of EAT1 was synthesized using optimized codons for E. coli genes ( http://www.kazusa.or.jp/codon/cgi-bin/spsearch.cgi?species=Escherichia+coli&c=s ) (sequence in Supplementary Table S3 ). EMSA analysis Full-length coding region of EAT1 fused with the maltose-binding protein tag was expressed in E. coli , using pMAL-c2X (NEB, USA). DNA fragments of the OsAP25 and OsAP37 promoters containing putative E-boxes were amplified by OsAP25-ChIP-F and OsAP25-ChIP-R, OsAP37-ChIP-F and OsAP37-ChIP-R, respectively, and cloned into pMD18-T (Takara, Dalian, China). Experimental procedures of qChIP-PCR and EMSA are as described in Xu et al. [7] Yeast cell-death measurement OsAP25 and OsAP37 full-length coding regions containing optimized codons for expression in bacteria, yeast and plants (sequences in Supplementary Table S3 , fused with c-MYC tag) were cloned into pESC-HIS (Agilent), using EcoR I and Spe I, and transformed into a YCA1-deficient stain, Δyca1 . Yeast caspase assays were carried out using the system developed by Madeo et al. [24] . Wild-type yeast cells (BY4741) were used as the control. For yeast cell-death assay, dead cells were stained by PI and examined using flow cytometry. Trypan blue staining of tobacco and Arabidopsis leaves Tobacco leaves were transfected by CAMV 35S-driven GFP , OsAP25-GFP , or OsAP37-GFP for transient expression of the proteins. 10 μM PepA-P (EMD Millipore, Billerica, USA) was injected into tobacco leaves with OsAP25-GFP or OsAP37-GFP . Forty-eight hours later tobacco leaves were collected, photographed and stained with Trypan blue. c-Myc-tagged OsAP25 and OsAP37 (with optimized codons for expression; sequences shown in Supplementary Table S3 ) were cloned into pER12 [50] using Age I and Xho I. The resulting constructs, OsAP25-pER and OsAP37-pER , are under the control of an inducible oestrogen receptor-based transactivator, XVW [50] . Fifteen-day-old Arabidopsis Col-0 and transgenic OsAP25-pER and OsAP37-pER seedlings were treated with estradiol and stained with Trypan blue 48 h after the treatment, as described by Coll et al. [28] Cell death on 80 leaves and 78 cotyledons were examined for each genotype. Plant transformation Transient expression in tobacco leaves was performed using the method by He et al. [51] Agrobacterium-mediated transformation of rice and Arabidopsis was performed as described by Hiei et al. [52] and Clough and Bent [53] , respectively. At least 10 independent transgenic lines for each construct were analysed. All primer sequences are listed in Supplementary Table S4 . Data deposition statement (accession numbers): OsAP25 , LOC_Os03g08790 ( http://www.gramene.org/ ) or Os03g0186900 ( http://rapdb.dna.affrc.go.jp/ ); OsAP37 , LOC_Os04g37570 or Os04g0448500; OsAP19 , LOC_Os02g27360 or Os02g0473200; MSP1 , LOC_Os01g68870 or Os01g0917500; GAMYB , LOC_Os01g59660 or Os01g0812000; UDT1 , LOC_Os07g36460 or Os07g0549600; TDR , LOC_Os02g02820 or Os02g0120500; PTC1 , LOC_Os09g27620 or Os09g0449000; API5 , LOC_Os02g20930 or Os02g0313400; OsCP1 , LOC_Os04g57490 or Os04g0670500. All of peptides included in the NJ tree were from NCBI. How to cite this article: Niu, N. et al. EAT1 promotes tapetal cell death by regulating aspartic proteases during male reproductive development in rice. Nat. Commun. 4:1445 doi: 10.1038/ncomms2396 (2013).